Three-dimensional view of ultrafast dynamics in photoexcited bacteriorhodopsin in the multiphoton regime and biological relevance 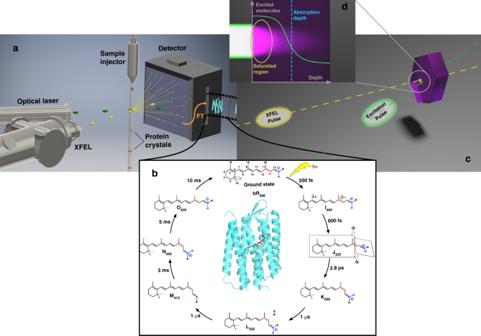Fig. 1: Making molecular movies and excitation considerations. aTime-resolved serial crystallography is schematically shown using a lipid cubic phase injector per ref.3. Femtosecond optical laser pulses (532 nm) initiate the photocycle in a train of bR crystals with random orientations. The fs X-ray (XFEL) pulses capture the photoinduced structural changes by diffraction that are Fourier Transformed (FT) to real space structures to make a movie of the structural changes.bThe photocycle of retinal in bacteriorhodopsin (bR) captured in the “molecular movie” film in the single photon regime (refer to text for details). Ground state bR (PDB code: 1C3W) is depicted in the center with retinal covalently bound to bR though a Schiff base linkage to a conserved lysine residue. The source of the transported proton is the protonated retinal Schiff base, highlighted in blue. The key isomerization step from all-transto 13-cisretinal occurs about the C13=C14 bond, accented in red.‡Subsequent, protein structural changes are occurring in the ps–ms time region in order to facilitate proton transport.cThe time base for the movies is determined by the speed of light and variable pathlength difference as shown between the fs excitation and fs X-ray probe pulses to give <100 fs time resolution to atomic motions.dThe inset shows the mismatch between the laser excitation, which is strongly absorbed, and the X-ray pulse, which samples the entire crystal thickness (10 µm scale). Excitation well above 1-photon per photoactive chromophore is often used to try to excite a larger fraction of the probed volume to decrease unexcited background scatter from obscuring the photoinduced structural changes. At such high fluences, saturation effects occur (shown) that also lead to fully resonant coherent 2-photon, sequential resonant 2-photon, nonresonant 2-photon, to n-photon transitions depending on the laser pulse width and associated peak power. Crystals on the order of the 1/eabsorption depth (dashed blue line) should be used for maximum contrast above background under conditions to ensure 1-photon absorption to well defined excited states (see text). 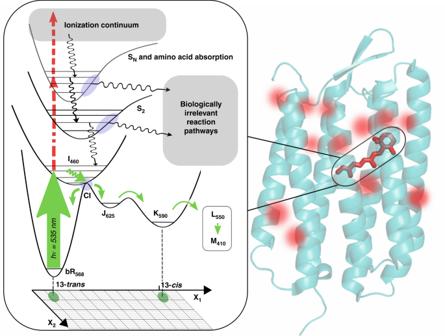Fig. 2: Photophysical and chemical pathways at high peak power and fluences. The seven transmembrane helical structure of bR is shown with retinal identified by the solid red structure. The red hot spots denote the positions for nonresonant two-photon excitation of Trp at high peak powers, which would be random and not contribute coherently to changes in diffraction (per ref.3). However, all the resonant multiphoton pathways involving retinal would occur at the same location in space, i.e. at the retinal site, and contribute to photoinduced changes in diffraction. The left panel shows the biologically relevant one-photon pathway (solid green) for photoisomerization of retinal in relation to the multiphoton pathways (dashed green). The functionally relevant motions are highly constrained by the protein structure in going from the initially formed photoisomer, which is strongly coupled to distinct retinal-protein conformational states (I-M). In contrast, the different multiphoton pathways to different excited state surfaces have relaxation channels (black wiggly arrows) to photoproducts in undefined reaction coordinate space (x1, x2) unrelated to biological function. The need to excite the biologically relevant one-photon pathway is clear. This figure shows the importance of exciting in the one-photon, linear response, regime (see text for guidelines). The most important aspect of this work is the rigor to which they characterized the excitation typically used in XFEL experiments. The authors studied not only the power dependence using multiple spectral markers to quantify nonlinear changes in photoproduct formation, but also determined the scattering (<20%) from their lipid cubic phase crystal delivery system. With the corrected incident fluence, they established that they used 36 photons per retinal within the 1/ e absorption length of the bR crystals. This detail alone clearly establishes that the experiments were conducted in the multiphoton regime. The corresponding peak power for their excitation pulse durations was 500 GW/cm 2 where the onset for nonlinear behavior occurs around 30 GW/cm 2 , in which case the initial state preparation is ill defined (see Fig. 2 of ref. [3] ). This finding has implications for all previous studies conducted using similar peak powers or fluences [5] , [6] , [7] , [8] , [9] . The authors made the case, based on theoretical calculations, that the clearly observed multiphoton processes in their peak power control studies were attributable to non-resonant two-photon absorption by the tryptophan (Trp) residues within the retinal binding site, i.e., the transition requires the simultaneous action of two photons at the excitation wavelength of 535 nm to have sufficient energy to excite Trp. This alone illustrates how high the peak power was. It was argued these excitation processes are inconsequential with respect to excitation of retinal. However, we estimate that the fully resonant 2-photon absorption of retinal at 535 nm is at least 2 orders of magnitude larger than the nonresonant process for Trp [10] , [11] . This estimate is further reinforced by the observed saturation of the non-resonant 2-photon absorption (800 nm) of retinal (bR) at 700 GW/cm 2 —to give a completely different photoproduct—that is specifically exploited for optical memory [12] , [13] . The fully resonant 2-photon absorption of retinal (at 535 nm) would saturate at more than an order of magnitude lower peak power than observed at 800 nm, approximately where the authors see the onset of nonlinear behavior (>30 GW/cm 2 , Fig. 2 of ref. [3] ), and lead to even higher multiphoton processes at higher powers. These resonant two-photon and higher processes of retinal access higher-lying electronic states, which can explore many different potential energy surfaces that lead to different photoproducts than the biologically relevant S 1 excited state channel (see Fig. 2 ). The most important fundamental point to come out of this work is that despite all the possible different photochemical pathways sampled from high lying electronic states accessed via multiphoton absorption, there is a remarkable convergence at long time (ms) to the previously assigned M structure [14] . It seems that no matter the starting point, the system is poised to channel energy into forming the structural intermediates most intimately involved in the key proton transfer step. This inadvertent discovery could end up being extremely important in trying to understand structure-function relationships of biological systems. It may well be that there is a multi-tiered optimization process at work. The surrounding protein matrix has clearly been optimized to selectively direct trans to cis isomerization at the C13-C14 position in the S1 excited state, which subsequently triggers a cascade of thermally sampled processes leading to proton translocation—the biological purpose for energy storage. There are still multiple, irrelevant, conformational pathways for both the retinal and surrounding protein possible at each step along the relaxation cascade that could negatively affect the water network and proton transport within the perturbed protein structure. There are many more substates and much longer time to sample such meandering pathways for the subsequent I to M intermediate steps than the ultrafast primary processes. There would need to be constraints on the fluctuations to keep the process focused as additional tiers of optimization. We may well be seeing our first evidence of just how strongly correlated the motions of the retinal and protein surroundings are to keep the reaction focused from femtoseconds to milliseconds. We would not have this insight without excessively “kicking” the retinal (via multiphoton processes) and still getting the same result as the biologically relevant excitation. There is, however, a caveat. The referenced “M” structure [14] was also determined using similarly high fluences, with >20 photons per retinal in the 1/ e absorption depth (Fig. 1d ), such that the total excess energy deposited into the protein by sequential multiphoton and associated temperature jump (order 100 °C, µs-ms decay) [15] , [16] will be comparable. In this case, this coincidence could be expected as a consequence of thermally sampled pathways—not photochemically driven. We will not be able to discern the level of organization and degree of dynamic coupling between the retinal and the protein structure until we determine the structural changes under biologically relevant conditions. To ensure one-photon processes to relevant excited states, the excitation fluence must be less than one photon per photoactive chromophore within the 1/ e absorption depth (ideally less than 0.2 photons to give <10% contribution from 2-photon channels), and normalized peak power dependences of transient spectra need to be done to confirm linear response (typically <100 GW/cm 2 ). It is the magnitude of the motions and correlations through space that define how the chemistry, in this case isomerization or a simple push, is transduced into biology. The pathway matters. This work is a significant step forward in putting us on the right track.